Correspondence: Reply to ‘The experimental requirements for a photon thermal diode’ 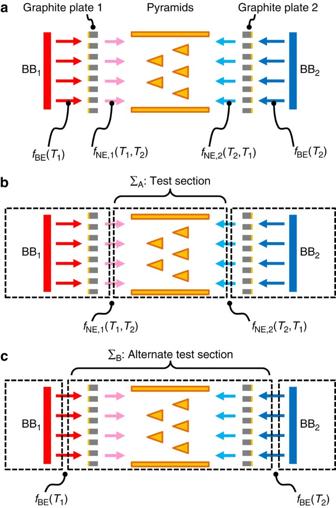Figure 1: Alternative analyses reveal a fundamental problem with the thermalizing graphite plate concept for inelastic thermal collimation. (a) Schematic of a configuration with proper symmetries1, using two mirror-imaged thermal collimators. The heat transfer response functionQ(T1,T2) can be analyzed using either of the control volumes depicted inb,c. (b) In the original work (for example, Supplementary Fig. 5c of ref.2), each graphite plate was considered part of its adjacent BB, corresponding to non-equilibrium reservoir boundary conditionsfNE,1(T1,T2) andfNE,2(T2,T1). (c) Alternatively, the graphite plates can be considered with the pyramids as ΣB. In this case, the reservoir boundary conditions are perfect blackbodies with equilibrium Bose-Einstein statisticsfBE(T1) andfBE(T2), analyzed further here inFig. 2. Clearly theQ(T1,T2) function must be the same whether calculated usingborc. 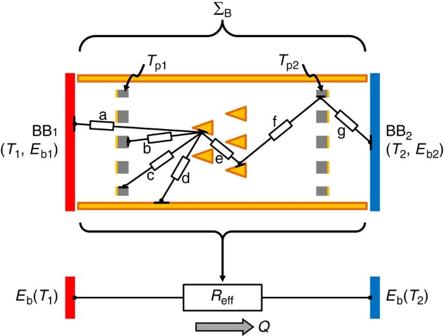Figure 2: Implications of a radiation resistor network analysis of ΣBfromFig. 1c. Top: All surfaces are discretized into differential areas and joined by numerous radiation resistors, a very few of which are indicated schematically as a–g. Each graphite plate has infinite thermal conductivity and thermalizes to its own unknown temperature (Tp1,Tp2), while the pyramids and test section sidewalls are taken as perfectly reflecting (diffuse and/or specular), and the two reservoirs as ideal BBs.Bottom: For these conditions, it is well known that the heat transfer analysis can be expressed as a linear system of equations4, corresponding to a single effective resistorReffbetween the driving potentialsEb1andEb2. Thus, the response functionQ(T1,T2) must be anti-symmetric upon the exchangeT1↔T2. We conclude that if it had used the correct two-plate symmetry as depicted here inFig. 1a, the thermalizing graphite plate scheme as originally conceived2could not rectify. How to cite this article: Chen, Z. et al . Correspondence: Reply to ‘The experimental requirements for a photon thermal diode’. Nat. Commun. 8 , 16136 doi: 10.1038/ncomms16136 (2017). Publisher’s note: Springer Nature remains neutral with regard to jurisdictional claims in published maps and institutional affiliations.